Imaging live cell in micro-liquid enclosure by X-ray laser diffraction Emerging X-ray free-electron lasers with femtosecond pulse duration enable single-shot snapshot imaging almost free from sample damage by outrunning major radiation damage processes. In bioimaging, it is essential to keep the sample close to its natural state. Conventional high-resolution imaging, however, suffers from severe radiation damage that hinders live cell imaging. Here we present a method for capturing snapshots of live cells kept in a micro-liquid enclosure array by X-ray laser diffraction. We place living Microbacterium lacticum cells in an enclosure array and successively expose each enclosure to a single X-ray laser pulse from the SPring-8 Angstrom Compact Free-Electron Laser. The enclosure itself works as a guard slit and allows us to record a coherent diffraction pattern from a weakly-scattering submicrometre-sized cell with a clear fringe extending up to a 28-nm full-period resolution. The reconstructed image reveals living whole-cell structures without any staining, which helps advance understanding of intracellular phenomena. Radiation damage is a serious problem in high-resolution microscopy, for example, electron microscopy or X-ray microscopy, which limits achievable resolution [1] , [2] . X-ray free-electron lasers (XFELs) can overcome the problem by freezing the sample in time using the femtosecond pulse duration instead of cryogenically cooling the sample [3] , [4] , [5] , [6] . Coherent X-ray diffraction (CXD) using XFELs thus has great potential for high-resolution imaging of biospecimens [7] , [8] . CXD has been developed using synchrotron radiation [9] , [10] and applied to high-contrast imaging of biological samples without the need for crystallization [11] , [12] , [13] , [14] , [15] , [16] , [17] , [18] , [19] . The femtosecond pulse duration of XFELs also has great potential to capture snapshots of biological samples close to its natural state. In this study, we use XFEL to observe living bacterial cells, Microbacterium lacticum ( M. lacticum ) [20] . Bacterial genetic information is generally contained in irregularly shaped nucleoids, which have stronger X-ray scattering power because of their phosphorus content [21] , [22] . M. lacticum , discovered in milk, is a heat-stable Gram-positive bacterium and is the type species of the genus [23] . Although contamination by thermoduric bacteria in raw milk is a severe agricultural problem [24] , little information is available about their cell biology because of their submicron size. M. lacticum has a typical rod shape but is much smaller than ordinary bacteria: it is about half the length and 10% of the volume as compared with Escherichia coli . Therefore, it is difficult to observe internal structures of the cell using conventional optical microscopy. We propose pulsed coherent X-ray solution scattering (PCXSS) using X-ray laser diffraction, which aims to achieve high-resolution imaging of biological samples in close-to-natural conditions. 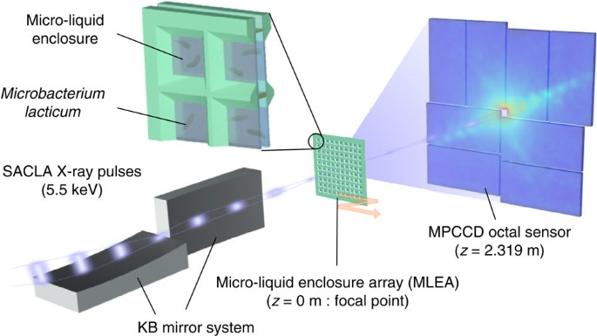Figure 1: PCXSS experiment for live cells. The XFEL beam from the SPring-8 Angstrom Compact Free-Electron Laser (SACLA) with a photon energy of 5.5 keV was focused at the sample position to a spot size of 1.5 μm × 2.0 μm using a Kirkpatrick-Baez (KB) mirror system27,28. An MLEA containing livingM. lacticumcells was placed in a vacuum in the MAXIC instrument. The MLEA was scanned to shoot each enclosure with a single XFEL pulse. Because the pulse duration of the XFEL beam was as short as ~10 fs, X-ray laser diffraction occurs before the sample is destroyed3,4,5,6. Single-shot CXD patterns were recorded with a multiport charge-coupled device (MPCCD) octal sensor29. Figure 1 shows the PCXSS experiment schematically. The key component of our PCXSS experiment is a micro-liquid enclosure array (MLEA) to keep biological samples in a solution close-to-natural conditions. The array structure is necessary in PCXSS experiments because the thin silicon nitride membranes, which separate the solution sample from the vacuum environment, are destroyed by a single XFEL pulse exposure. Similar liquid enclosures have been used to image biological samples in solution with scanning transmission electron microscopy [25] and CXD microscopy [26] . XFEL can further resolve the radiation damage problem for biological samples in solution. We perform PCXSS measurement to observe living M. lacticum cells in MLEA chips and successfully reveal the internal structures. Figure 1: PCXSS experiment for live cells. The XFEL beam from the SPring-8 Angstrom Compact Free-Electron Laser (SACLA) with a photon energy of 5.5 keV was focused at the sample position to a spot size of 1.5 μm × 2.0 μm using a Kirkpatrick-Baez (KB) mirror system [27] , [28] . An MLEA containing living M. lacticum cells was placed in a vacuum in the MAXIC instrument. The MLEA was scanned to shoot each enclosure with a single XFEL pulse. Because the pulse duration of the XFEL beam was as short as ~10 fs, X-ray laser diffraction occurs before the sample is destroyed [3] , [4] , [5] , [6] . Single-shot CXD patterns were recorded with a multiport charge-coupled device (MPCCD) octal sensor [29] . Full size image 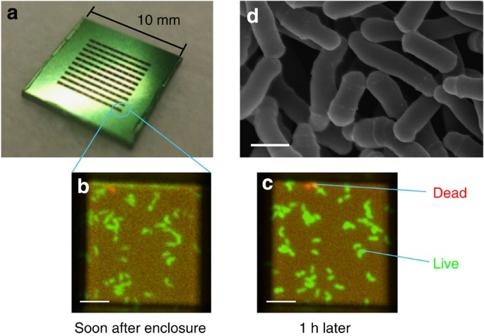Figure 2: MLEA and live-dead experiment. (a) MLEA can retain biological samples in a solution between two thin silicon nitride membranes, which separate the solution sample from a vacuum environment. In the current design, a single 10 mm × 10 mm MLEA chip contains a 10 × 10 array of enclosures. (b,c) Live-dead experiment was performed to confirm that the MLEA can preserve live cells long enough to perform a PCXSS measurement (Methods). The fluorescence microscopy images show live cells in green and dead cells in red and were taken soon after enclosure (b) and 1 h after enclosure (c). During the 1 h interval, MLEA was placed in a vacuum environment to simulate PCXSS measurement. The experiment showed that 99% of the cells are alive in MLEAs at 1 h after enclosure. Scale bars: 5 μm (inbandc). (d) A scanning electron microscopy (SEM) image ofM. lacticum cellsshows the typical shapes and sizes (Methods). Scale bar: 500 nm (ind). Live cells in MLEA Figure 2a shows an MLEA chip we developed. We enclosed M. lacticum cells in MLEA and observed under fluorescence microscope ( Fig. 2b,c ). In the fluorescence microscopy study, live cells are labelled in green and the dead ones in red (Methods). Our experiment revealed that 99% of the cells are alive in MLEAs at 1 h after enclosure being placed in a vacuum environment. Note here that no fluorescent labelling was applied to the samples used in the PCXSS measurement. We also verified that each enclosure remained tightly sealed and retained the solution sample, even when an adjacent enclosure was broken in a vacuum environment. Figure 2d shows a scanning electron microscopy (SEM) image of M. lacticum cells for reference. Figure 2: MLEA and live-dead experiment. ( a ) MLEA can retain biological samples in a solution between two thin silicon nitride membranes, which separate the solution sample from a vacuum environment. In the current design, a single 10 mm × 10 mm MLEA chip contains a 10 × 10 array of enclosures. ( b , c ) Live-dead experiment was performed to confirm that the MLEA can preserve live cells long enough to perform a PCXSS measurement (Methods). The fluorescence microscopy images show live cells in green and dead cells in red and were taken soon after enclosure ( b ) and 1 h after enclosure ( c ). During the 1 h interval, MLEA was placed in a vacuum environment to simulate PCXSS measurement. The experiment showed that 99% of the cells are alive in MLEAs at 1 h after enclosure. Scale bars: 5 μm (in b and c ). ( d ) A scanning electron microscopy (SEM) image of M. lacticum cells shows the typical shapes and sizes (Methods). Scale bar: 500 nm (in d ). Full size image PCXSS experimental setup We performed PCXSS experiments using the SPring-8 Angstrom Compact Free-Electron Laser (SACLA) [27] (Methods). The XFEL pulses from the SACLA with a photon energy of 5.5 keV, a pulse duration of ~10 fs and a repetition rate of 10 Hz were coherently focused to a 1.5 μm × 2.0 μm spot size [28] . The focused XFEL beam illuminated the sample in an MLEA that was contained in a Multiple Application X-ray Imaging Chamber (MAXIC). Single-shot CXD patterns were recorded with a multiport charge-coupled device (MPCCD) octal sensor [29] located 2.319 m downstream from the sample. The MPCCD has 2048 × 2048 pixels with a pixel size of 50 μm × 50 μm. When using MLEAs, the amount of sample required per XFEL shot does not depend on the repetition rate of XFEL in contrast to continuous sample injection schemes [5] , [6] , where samples are wasted in the intervals between XFEL pulses. Therefore, MLEA can bring great benefit to maintain a high efficiency of sample utilization even with a low repetition rate of SACLA. Background scattering reduction by MLEA In a CXD experiment, it is essential to reduce background scattering for high-quality data acquisition. In our PCXSS experiment, MLEA containing saline solution produced lower background scattering than the case without MLEA ( Fig. 3 ); the window frame of each enclosure with an aperture size of ~20 μm acts as a guard slit and helps reduce parasitic scattering from upstream components. In addition, because the XFEL beam enters and exits perpendicular to the flat surfaces of enclosure windows, uniform phase-advance occurs but no parasitic scattering is generated in principle. The thickness of the MLEA solution layer can be controlled precisely by using a nanometre-scale spacer. It is ideal to make the solution layer slightly thicker than the sample size to minimize background scattering from the solvent. In our experiment, we set the solution layer to 500 nm to match M. lacticum dimensions, which have a rod shape with ~200 nm in diameter and 500–1,000 nm in length ( Fig. 2d ). 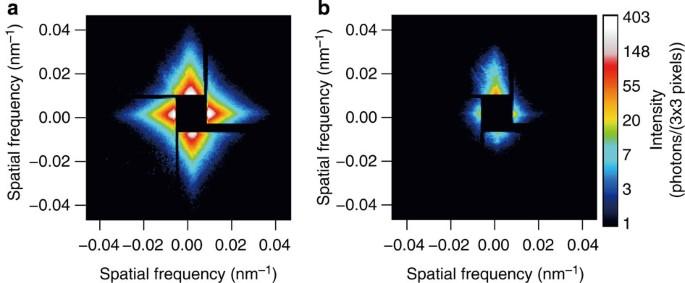Figure 3: Reduction of background scattering by MLEA window frame. (a) Scattering pattern when nothing was placed at the focal plane. (b) Scattering pattern from saline solution (NaCl 0.9% (w/v)) in MLEA with a solution layer thickness of 500 nm.aandbare shown in a logarithmic scale. The average of 73 shots for each case is shown. The maximum photon counts per pixel for the averaged scattering patterns are 452 foraand 45 forb, and the reduction rate is 9.9%. The average photon counts per pixel are 3.5 foraand 0.5 forb, and the reduction rate is 14.4%. The result demonstrates that the frame of the MLEA window helped reduce parasitic scattering. The average incident pulse energies measured at the optics hutch downstream of the double total-reflection mirrors are 203 and 195 μJ per pulse foraandb, respectively. Note that X-ray absorption is negligible forbwith a transmission of 98% for 5.5 keV X-rays. Figure 3: Reduction of background scattering by MLEA window frame. ( a ) Scattering pattern when nothing was placed at the focal plane. ( b ) Scattering pattern from saline solution (NaCl 0.9% (w/v)) in MLEA with a solution layer thickness of 500 nm. a and b are shown in a logarithmic scale. The average of 73 shots for each case is shown. The maximum photon counts per pixel for the averaged scattering patterns are 452 for a and 45 for b , and the reduction rate is 9.9%. The average photon counts per pixel are 3.5 for a and 0.5 for b , and the reduction rate is 14.4%. The result demonstrates that the frame of the MLEA window helped reduce parasitic scattering. The average incident pulse energies measured at the optics hutch downstream of the double total-reflection mirrors are 203 and 195 μJ per pulse for a and b , respectively. Note that X-ray absorption is negligible for b with a transmission of 98% for 5.5 keV X-rays. Full size image CXD patterns from live cells We succeeded in recording CXD patterns from intact M. lacticum cells with single XFEL pulses ( Fig. 4 , Supplementary Fig. 1 ). A few percent of recorded data indicate hitting M. lacticum cells, and a few tens of percent of the hits are likely from a single cell (see Methods for more details on the measurement efficiency). We consider that the low hit rate is due to gravitational settling, and it can be improved by, for example, immobilizing cells using silicon nitride membranes coated with polylysine [30] , [31] . Note that gravitational settling does not occur for smaller-sized particles where diffusion due to Brownian motion becomes dominant over the gravitational effect (Methods). 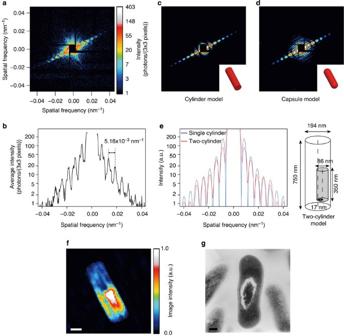Figure 4: Experimental CXD pattern and reconstruction. (a) Measured CXD pattern from a liveM. lacticumcell. (b) Line profile in the fringe direction of the measured CXD pattern. (c,d) Simulated CXD patterns in the cylinder (c) and capsule (d) models (Methods). Corresponding 3D structures with Euler angles (28°, −40°, 0°) are shown in the lower panels. (e) Line profiles of the simulated CXD patterns in the fringe direction in the single-cylinder (blue) and the two-cylinder (red) models (Methods). The fringe visibility degrades in the two-cylinder model as compared in the single-cylinder model. (f) Reconstructed image of anM. lacticumcell. (g) TEM image of anM. lacticumcell.a–eare shown in a logarithmic scale;fandgare shown in a linear scale. Scale bars: 100 nm (infandg). Figure 4: Experimental CXD pattern and reconstruction. ( a ) Measured CXD pattern from a live M. lacticum cell. ( b ) Line profile in the fringe direction of the measured CXD pattern. ( c , d ) Simulated CXD patterns in the cylinder ( c ) and capsule ( d ) models (Methods). Corresponding 3D structures with Euler angles (28°, −40°, 0°) are shown in the lower panels. ( e ) Line profiles of the simulated CXD patterns in the fringe direction in the single-cylinder (blue) and the two-cylinder (red) models (Methods). The fringe visibility degrades in the two-cylinder model as compared in the single-cylinder model. ( f ) Reconstructed image of an M. lacticum cell. ( g ) TEM image of an M. lacticum cell. a – e are shown in a logarithmic scale; f and g are shown in a linear scale. Scale bars: 100 nm (in f and g ). Full size image X-ray scattering from a submicrometre-sized M. lacticum is weak and is comparable in intensity to the background scattering without MLEA shown in Fig. 3a . This implies that the background scattering reduction effect of MLEA demonstrated in Fig. 3b was essential to the successful recording of the CXD pattern from an M. lacticum . The dose applied to the cell was estimated to be ~100 MGy from an XFEL pulse energy of ~60 μJ at the sample position. Note that even highly radiation-resistant Deinococcus radiodurans cannot survive at 20 kGy in conventional imaging methods [32] . Numerical simulation of CXD patterns The CXD pattern in Fig. 4a contains a clear fringe extending in one direction. The fringe spacing and orientation indicates a sample width of 194 nm and is tilted by 28°. The width is comparable to the diameter of an M. lacticum cell. The full-period resolution estimated from the highest scattering angle of the fringe is 28 nm ( Fig. 4b ). Although a CXD pattern from a two-dimensional rectangular object generally produces fringes extending in two directions perpendicular to each other, CXD patterns simulated with three-dimensional cylinder and capsule models typically produce a fringe that extends in one direction ( Fig. 4c,d , Supplementary Fig. 2 , Methods ); a fringe cannot be observed when it does not intersect the Ewald sphere in 3D reciprocal space. When multiple samples are present under an illuminated volume, fringes should appear in multiple directions ( Supplementary Figs 1a, 2b ). The above considerations strongly indicate that the experimental CXD pattern originates from a single M. lacticum cell. In addition, the reduced fringe visibility observed in Fig. 4b has a close relation to the intracellular structure ( Fig. 4e , Methods). The simulations above also suggest the possibility of 3D modelling from a single-shot CXD pattern when the sample structure can be parameterized with a simple model. Image reconstruction We performed image reconstruction from the experimental CXD pattern shown in Fig. 4a by using the relaxed averaged alternating reflections (RAAR) algorithm [33] , the noise-tolerant hybrid input-output (HIO) algorithm [34] and the shrink-wrap algorithm [35] (Methods). Figure 4f shows the reconstructed image of an M. lacticum cell. It is rod shaped with a width and length of ~194 nm and ~570 nm, respectively, which agreed well with the known shape and size of M. lacticum cells. To test the consistency of the reconstruction, we performed two independent image reconstruction runs using different initial random seeds, and the result in Supplementary Fig. 3 shows the small dependence of reconstruction on initial phases. Full-period spatial resolution of the reconstructed image in the fringe direction was estimated to be ~37 nm ( Fig. 5 ) [12] , [36] . 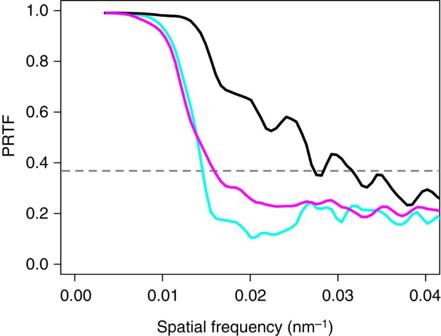Figure 5: Estimation of resolution using phase-retrieval transfer function. Phase-retrieval transfer function (PRTF)12,36for the reconstructed image shown inFig. 4faveraged over whole shells of the same spatial frequency (magenta line). PRTF averaged over shells within ±15° around the fringe direction (black line), and that averaged over shells within ±15° around the direction perpendicular to the fringe (turquoise line) are also drawn. Figure 5: Estimation of resolution using phase-retrieval transfer function. Phase-retrieval transfer function (PRTF) [12] , [36] for the reconstructed image shown in Fig. 4f averaged over whole shells of the same spatial frequency (magenta line). PRTF averaged over shells within ±15° around the fringe direction (black line), and that averaged over shells within ±15° around the direction perpendicular to the fringe (turquoise line) are also drawn. Full size image We recorded a single-shot CXD pattern of a live M. lacticum cell in MLEA using SACLA, and successfully reconstructed the cell image ( Fig. 4f ). It is remarkable that the internal density is non-uniformly distributed throughout the cell. The strong image-intense region in the lower area of the cell is dumbbell shaped, with two islands composed of high intensity and moderately high intensity regions, coloured in white and red, respectively. In the upper area of the cell, non-uniform density is also observed within a weak intensity region. The lower area of the cell may contain highly electron-dense materials, such as DNA molecules. In fact, the image intensity difference between the upper and lower regions of the cell can be roughly explained by assuming that they are mostly composed of protein and nucleic acids, respectively [37] . Note that the reconstructed image shows the contrast between the sample and the solvent. The image resembles the transmission electron microscopy (TEM) image shown in Fig. 4g . It should be stressed here that the X-ray image was obtained for an unstained living cell, while the TEM image was for a chemically fixed ultrathin section stained with uranyl acetate and lead citrate. Our experiment demonstrated that whole-cell imaging by the proposed PCXSS method can reveal the natural structures of live cells at the nanoscale without any staining, which have been inaccessible by other methods. The results of this research will potentially create a breakthrough in whole-cell biology. For example, the presently achieved resolution, which far exceeds conventional optical microscopy, could provide clues towards understanding nucleoid structures in living cells. Multiple snapshot images could also reveal the dynamics of important cellular events, such as genome replication and subsequent cell division. The method is also applicable to imaging biomolecules in solution. Important targets include supramolecular complexes, multiple complexes and intrinsically disordered proteins, which are difficult to crystallize. To realize biomolecular imaging with PCXSS, a huge enhancement in the CXD signal is required. A straightforward way to increase the CXD signal is to intensify the XFEL beam by advances in accelerator or X-ray optics technologies [38] . Another way is to enhance the number of scatterers by illuminating many copies of a molecule in solution. In the latter case, speckled scattering patterns can be obtained with highly-focused XFELs because neither ensemble averaging nor time averaging occurs in contrast to conventional X-ray solution scattering [39] . There are different strategies to obtain structural information from speckled scattering patterns from many copies: one is to perform single-particle analysis as practiced in electron microscopy to obtain 3D structures from projection images of many particles in random orientations [40] , [41] ; another way is to numerically retrieve single-particle CXD data from the scattering patterns of many copies [42] , [43] , [44] . The PCXSS method will also offer insights for protein dynamics by revealing metastable conformations of molecules in solution. Preparation of bacterial cells The M. lacticum NBRC14135 T strain was obtained from the Biological Resource Center (NBRC), National Institute of Technology and Evaluation, Kisarazu, Japan. Cells were grown at 37 °C with shaking in medium containing 1% (w/v) tryptone (Becton Dickinson and Company, Sparks, MD), 0.5% (w/v) Bact Yeast Extract (Becton Dickinson and Company, Sparks, MD) and 0.5% (w/v) NaCl, pH 7.0 and were stored in a Microbank (PRO-LAB, Round Rock, TX) at −80 °C until use. Cells were subcultured in 200 ml of the culture medium and incubated at 37 °C for 16 h. Cells were collected by centrifugation after filtration through a 1-μm Glass Fibre Membrane (PALL, Port Washington, NY) to remove fine dust contamination in the growth medium. Cells were suspended in 0.9% (w/v) NaCl, which had been filtered through a DISMIC-25 cs disposable syringe filter unit (Advantec, Tokyo, Japan). Colony-forming units (CFUs) were determined by counting colony numbers on 1.5% (w/v) agar medium plates, inoculated with 100-μl aliquots of cultures grown for 2 days at 37 °C. Live-dead experiment of bacterial cells in MLEA Approximately 1 × 10 11 CFU per ml of M. lacticum cells in 10 μl of 0.9% (w/v) NaCl were treated with the LIVE/DEAD BacLight Bacterial Viability Kit (Invitrogen), preincubated for 10 min at 4 °C and then enclosed in an MLEA chip. During incubation for 1 h at 25 °C, the MLEA chip was placed in a vacuum of 10 −3 Pa to simulate conditions during the PCXSS experiment. The ratio of living and dead cells was determined by counting the green (live) and red (dead) fluorescent cells on photographs obtained by fluorescence microscopy (Olympus BX51). PCXSS experiment The PCXSS experiment for live M. lacticum cells was performed using BL3 of SACLA [27] . The XFEL beam from the SACLA had a photon energy of 5.5 keV, a pulse duration of ~10 fs and a repetition rate of 10 Hz. The average pulse energy of the beam was 260 μJ per pulse just after the undulator. Higher harmonic X-rays were reduced using double total-reflection mirrors in the optics hutch and guided to the experimental stations. In the third experimental station, the beam was focused by a Kirkpatrick-Baez mirror system to a spot size of 1.5 μm × 2.0 μm (full-width at half maximum) [28] at the sample position in the MAXIC instrument. The MAXIC instrument in a vacuum of ~10 −3 Pa contains two sets of cross slits, which reduce parasitic scattering from upstream components, and MLEA chips in the focal plane. Each MLEA chip retains a 2-μl aliquot of M. lacticum cells in 0.9% (w/v) NaCl with a cell concentration of ~1 × 10 10 CFU per ml at ~25 °C. MLEA chips mounted on motorized stages were scanned to shoot each enclosure with a single pulse. We aligned the MLEA chip to the XFEL beam by using a retractable on-axis zoom lens camera to observe the sample. For alignment, we first expose the Silicon frame of an MLEA chip with a single XFEL pulse and mark the damaged spot position on the monitor screen of the zoom lens camera. By using the mark on the monitor screen, we determined the coordinates of each enclosure without exposing it to the XFEL beam. Single-shot CXD patterns from live M. lacticum cells were recorded with an MPCCD octal sensor [29] , having 2,048 × 2,048 pixels with a pixel size of 50 μm × 50 μm, located 2.319 m downstream from the sample. The sensor has single-photon sensitivity with a system noise of ~300 electrons at an operating temperature of −30 °C, which corresponds to ~0.2 photons for 5.5 keV X-rays. The variable-size aperture at the centre of the sensor through which the direct beam may pass was set at 3.5 mm. The line profile of the measured CXD pattern shown in Fig. 4b was computed by averaging the diffraction intensities over a width of ±0.0016, nm −1 , which corresponds to the width of the central speckle originated from an object with a length of ~600 nm. The full-period resolution estimated from the highest scattering angle of the fringe (spatial frequency of 0.035 nm −1 ) is ~28 nm with a threshold of two photons per 3 × 3 pixels. The threshold was determined by considering a background intensity of 0.46±0.92 photons per 3 × 3 pixels far from the fringe. Statistical information about the measurement A single MLEA chip contains a 10 × 10 array of enclosures. Each enclosure was exposed to a single XFEL pulse. Among 100 single-shot data recorded for a single 10 × 10 array MLEA chip, we observed a few coherent diffraction patters indicative of hitting M. lacticum cells, and a few tens of percent of the hits are likely from a single cell, although it is difficult to count them precisely for weak diffraction data of submicrometre-sized unstained biospecimens. We consider that the low hit rate is due to gravitational settling, which does not occur for smaller-sized particles where diffusion due to Brownian motion becomes dominant over the gravitational effect. In fact, for gold nanoparticle self-assemblies with a size of ~100 nm, the probability of hitting sample was increased to a few tens of percent, an order of magnitude larger than for M. lacticum cells. According to ref. 45 , the probability of hitting single soot particles injected using an aerosol sample injector [5] , [45] , [46] is 0.07%. In femtosecond serial crystallography using a liquid jet sample injector [6] , [47] , the probability of recording indexable diffraction patterns was reported to be 3% in ref. 47 . Here, liquid jet sample injectors have been used for crystalline samples only, where Bragg diffraction is dominant over background scattering from the liquid jet. MLEA chips can be also usefully applied to micro- and nano-crystals. Here, shadowing of diffracted X-rays by the MLEA substrate limits the maximum scattering angle recordable to ~55°, when (100) silicon substrates with anisotropic wet-etching is used in MLEA chips. In our current measurement system, data acquisition rate is very low because of the slow movement of the sample stages. It takes 3 s to move an MLEA chip to the adjacent enclosure with an interval of 600 μm and 417 s to complete a raster scan of a 10 × 10 array MLEA chip. The hit rate of our measurement is ~0.005 particle diffraction patterns per second. It is technically feasible to develop fast sample stages in synchronization with the XFEL pulses for a relatively low repetition rate of, for example, SACLA. In container-free sample injection schemes, data acquisition has been already performed in synchronization with the XFEL pulses, and higher hit rate is achieved. For example, a hit rate of ~0.05 particle diffraction patterns per second has been reported for an aerosol sample injector [45] , [46] and four indexable diffraction patterns per second for a liquid jet sample injector [47] . There is also room for improvement in the sample exchange scheme. In our current system, we have to vent the entire chamber of the MAXIC instrument in exchanging samples. In recent measurement, we recorded ~10 4 single-shot data in two days of beamtime. A fast sample exchange scheme in addition to fast sample stages mentioned above will make the measurement much more efficient. Image reconstruction Image reconstruction was carried out in two steps on the experimental CXD pattern shown in Fig. 4a after centrosymmetrization. In the first step, the support area was refined using RAAR [33] with shrink-wrap [35] (2,000 steps) and subsequent noise-tolerant HIO [34] with the fixed support (1,000 steps). We set the initial support to have a rectangular shape with a tilt angle of 28° as determined from the fringe direction. The initial support size was set to 270 nm in width and 1.2 μm in length. The feedback parameter β was set to 0.87 and the support was updated every 50 iterations with a threshold of 0.05. We initially set the kernel of the shrink-wrap algorithm to 3 pixels and gradually reduced it to 1.5 pixels after 2,000 iterations. Using the results with 5,000 different initial random seeds, 2,891 good quality images with smaller reconstruction-errors were selected, and the new support was estimated by majority. In the refinement of the support, the reconstructed images were aligned with each other using the correlation coefficient ( c.c. ) defined by where { t p,q } and { r p,q } are the electron densities of two reconstructed images. Possibility of image inversion is also considered here. The refined support has a width and length of ~225 nm and ~612 nm, respectively. In the second step, image reconstruction was performed using RAAR [33] (1,000 steps) and subsequent noise-tolerant HIO [34] (1,000 steps) with the fixed support. The feedback parameter β was set to 0.87 for both algorithms. Using the results with 5,000 different initial random seeds, 119 images with high similarity ( c.c . with a representative>0.94) were selected and averaged. Finally, we obtained a rod-shaped image with a width and length of ~194 nm and ~570 nm, respectively ( Fig. 4f ). Numerical simulation of CXD patterns Supplementary Fig. 2 shows CXD patterns simulated using cylinder and capsule models in several orientations specified by Euler angles. The definition of the Euler angles is explained in Supplementary Fig. 2c . The cylinder has a diameter and height of 194 nm and 750 nm, respectively. The capsule consists of one cylinder, having a diameter and height of 194 nm and 550 nm, respectively, and two hemispheres (caps) with diameters of 194 nm. The object with a height of 750 nm produces a projection image with a height of ~600 nm for an Euler angle of (28°, −40°, 0°). In this orientation, the object can fit within the solution layer of MLEA with a depth of ~500 nm. Parameters in the PCXSS experiment were used in the simulation. CXD patterns for the cylinder model with uniform electron-density distribution were computed using an analytical formula. CXD patterns for the capsule model were simulated using 100,000 pseudo-particles distributed randomly and uniformly inside the capsule. Each pseudo-particle has a Gaussian electron-density distribution with a s.d. of 3.6 nm. The Euler angles for the two-capsule simulation shown in Supplementary Fig. 2b are (28°, −40°, 0°) and (−40°, 30°, 0°), respectively, and the translational vector between the two centres is (400 nm, −200 nm, 0 nm). Figure 4e demonstrates the degradation of fringe visibility using a two-cylinder model. The model structure consists of the external cylinder, having a diameter and height of A and H , respectively, and the internal cylinder, having a diameter and height of a and h , respectively. The two cylinders are separated by t =( t x , t y, t z ). Line profile of the CXD pattern in the fringe direction simulated in the two-cylinder model for Euler angles of ( φ , θ ,0) is computed analytically as where C , ρ ex and ρ in are a constant, the electron densities of the external and internal cylinders, respectively. J 1 ( x ) is the first order Bessel function. It is noted that the line profile does not depends on ( t y, t z ), nor the Euler angles of the model. ρ in / ρ ex is set to be 2.5. SEM and TEM measurements For the SEM measurement, a JEOL JSM-6320F electron microscope was used at an accelerating voltage of 5 kV; M. lacticum cells were fixed with glutaraldehyde and osmium tetroxide, dried by the critical point method and coated with an osmium plasma coater. For the TEM measurement, a JEOL JEM-1200EX electron microscope was used at an accelerating voltage of 80 kV; M. lacticum cells were fixed with glutaraldehyde and osmium tetroxide, dehydrated with ethanol and embedded in epoxy resin (EPON812) at 60 °C; an ultramicrotome was then used to produce 80–90 nm-thick sections; the sections were stained with uranyl acetate and lead citrate, and coated with carbon. Sample preparation and measurement of SEM and TEM were performed by Hanaichi UltraStructure Research Institute through an agent of Filgen, Inc. How to cite this article: Kimura, T. et al. Imaging live cell in micro-liquid enclosure by X-ray laser diffraction. Nat. Commun. 5:3052 doi: 10.1038/ncomms4052 (2014).